The neuropeptide NLP-22 regulates a sleep-like state inCaenorhabditis elegans Neuropeptides have central roles in the regulation of homoeostatic behaviours such as sleep and feeding. Caenorhabditis elegans displays sleep-like quiescence of locomotion and feeding during a larval transition stage called lethargus and feeds during active larval and adult stages. Here we show that the neuropeptide NLP-22 is a regulator of Caenorhabditis elegans sleep-like quiescence observed during lethargus. nlp-22 shows cyclical mRNA expression in synchrony with lethargus; it is regulated by LIN-42, an orthologue of the core circadian protein PERIOD; and it is expressed solely in the two RIA interneurons. nlp-22 and the RIA interneurons are required for normal lethargus quiescence, and forced expression of nlp-22 during active stages causes anachronistic locomotion and feeding quiescence. Optogenetic stimulation of the RIA interneurons has a movement-promoting effect, demonstrating functional complexity in a single-neuron type. Our work defines a quiescence-regulating role for NLP-22 and expands our knowledge of the neural circuitry controlling Caenorhabditis elegans behavioural quiescence. Neuropeptides are central to mechanisms by which biological clocks temporally align animal behaviour with recurring internal or external conditions. In mammals, the neuropeptide hypocretin/orexin is secreted from lateral hypothalamic neurons to promote wakefulness during the optimal time of day for foraging [1] . Other mammalian neuropeptides shown or proposed to regulate behavioural outputs of circadian clocks include prokineticin [2] , epidermal growth factor (EGF) [3] , neuropeptide S [4] , prolactin-releasing peptide [5] , urotensin II [6] and neuromedin S [7] . In the fruit fly Drosophila melanogaster , the neuropeptide pigment-dispersing factor (PDF) is released from central nervous system circadian neurons to control sleep/wake behaviour [8] , [9] , [10] , emphasizing a conserved role for neuropeptides in translating clock information to behaviour [8] . In Caenorhabditis elegans (C. elegans), sleep-like behaviour is observed during lethargus periods, which occur at transitions between each of the four larval stages and between the fourth larval stage and the adult stage [11] . During lethargus, animals, cease locomotion, feeding and foraging, are less responsive to stimuli and display a homoeostatic response to forced movement [12] , [13] . Signalling pathways involving cAMP-dependent protein kinase (PKA), cyclic GMP-dependent protein kinase (PKG), EGF and PDF, which have roles in the regulation of mammalian and/or Drosophila sleep, also function in the regulation of C. elegans sleep-like quiescence [12] , [14] , [15] , suggesting that C. elegans quiescence has fundamental similarities to sleep in other animals. Additional molecular similarity between quiescence during lethargus and mammalian sleep is demonstrated by the larval cycling of expression of the protein LIN-42, which is homologous to the core circadian protein PERIOD [16] . lin-42 is required for proper timing of lethargus [17] , much as period is required for proper timing of circadian sleep [18] , but mechanisms by which lin-42 may affect quiescent behaviour were previously unknown. Here we identify the gene nlp-22 as a lin-42 -regulated gene affecting quiescent behaviour. nlp-22 encodes a neuropeptide whose function and expression were previously unknown. We show that nlp-22 can induce quiescence in normally active animals and is necessary for normal lethargus quiescence. In addition, we present evidence of a surprising functional complexity of neurons expressing NLP-22. Our findings expand our knowledge of the neural circuitry controlling C. elegans behavioural quiescence. nlp-22 expression cycles in response to a larval clock The activity of many mammalian neuropeptides with roles in clock regulation is controlled at the level of mRNA abundance. We therefore reasoned that a somnogenic peptide controlled by the larval clock would be upregulated before or during lethargus. We performed a transcriptional profiling experiment (manuscript in preparation) in precisely staged animals to identify genes with elevated expression before or during the fourth lethargus stage. mRNA abundance of the gene nlp-22, which encodes a protein predicted to be processed into a neuropeptide [19] , was higher in the L4 stage than in lethargus. Using qRT–PCR, we confirmed that nlp-22 mRNA expression cycles with a constant phase relationship to lethargus ( Fig. 1a ). nlp-22 mRNA peaked midway through the active larval stages, decreased during each lethargus stage, and was absent in adults. 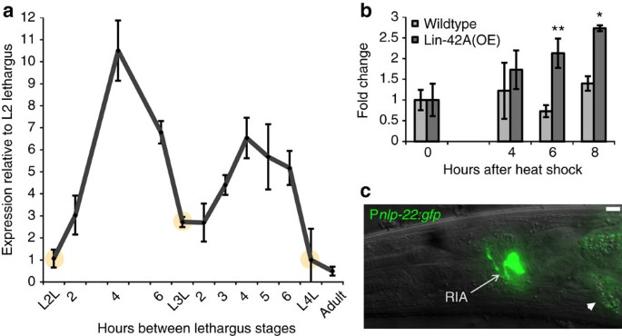Figure 1:nlp-22is expressed in a dynamic manner in the RIA interneurons. (a) mRNA expression during larval development. Expression levels cycle in synchrony with each lethargus stage. Yellow circles depict each lethargus stage, as defined by cessation of feeding of the animals (Biological replicates per time point ≥3, technical replicates=2 for each biological replicate; error bars represent s.e.m.). (b)nlp-22expression is increased in response tolin-42overexpression during the adult stage. (*P<0.05, **P<0.005, Student’s two-tailedt-test, biological replicates per condition ≥5, technical replicates=2 for each biological replicate; error bars represent s.e.m.). (c) Annlp-22transcriptional GFP reporter is expressed in the RIA neurons (arrow). Intestinal auto-fluorescence is also observed (arrow head). Scale bar=5 μM. Figure 1: nlp-22 is expressed in a dynamic manner in the RIA interneurons. ( a ) mRNA expression during larval development. Expression levels cycle in synchrony with each lethargus stage. Yellow circles depict each lethargus stage, as defined by cessation of feeding of the animals (Biological replicates per time point ≥3, technical replicates=2 for each biological replicate; error bars represent s.e.m.). ( b ) nlp-22 expression is increased in response to lin-42 overexpression during the adult stage. (* P <0.05, ** P <0.005, Student’s two-tailed t -test, biological replicates per condition ≥5, technical replicates=2 for each biological replicate; error bars represent s.e.m.). ( c ) An nlp-22 transcriptional GFP reporter is expressed in the RIA neurons (arrow). Intestinal auto-fluorescence is also observed (arrow head). Scale bar=5 μM. Full size image Given the cyclical nature of nlp-22 expression, we hypothesized that NLP-22 signalling is regulated by the larval clock. The C. elegans orthologue of the core circadian regulator PERIOD is LIN-42, which is required for the synchronization of lethargus quiescence and moulting [16] , [17] . Like PERIOD, which shows cyclical expression with a circadian periodicity in insects and mammals [20] , LIN-42 shows cyclical expression with larval periodicity in C. elegans [16] , [21] . LIN-42 expression has a similar phase relationship to lethargus as NLP-22. We found that LIN-42A anachronistic overexpression induced an increase in nlp-22 mRNA ( Fig. 1b ), suggesting that nlp-22 transcription is downstream of a larval lin-42 -based clock. nlp-22 is expressed in the pair of RIA interneurons To determine where nlp-22 is expressed, we generated a transcriptional reporter by placing green fluorescent protein (GFP) under the control of nlp-22 regulatory DNA. We observed expression only in one pair of head neurons, which we identified as the RIA interneurons, based on process morphology and in comparison with the expression of the previously characterized gene glr-3 ( Fig. 1c and Supplementary Fig. S1a ). Thus, nlp-22 expression is cyclical and restricted to the RIA neurons. NLP-22 is predicted to be secreted [19] . Secreted proteins in C. elegans , when fused to a fluorescent moiety on their C-terminus, can be visualized in cells outside of the cells in which they are expressed [22] . When we fused GFP to the C-terminus of the NLP-22 preproprotein, we observed green fluorescence in several neurons in the head as well as in the ventral nerve cord ( Supplementary Fig. S1b ), supporting the notion that NLP-22 is a secreted peptide. When we fused GFP to the N-terminus of the NLP-22 preproprotein, expression was exclusively in the RIA neurons, presumably because the GFP protein interfered with the functionality of the signal sequence ( Supplementary Fig. S1c ). Thus, our data indicate that the NLP-22 peptide is processed and secreted from the RIA interneurons and may be acting by synaptic and/or neuroendocrine mechanisms. NLP-22 induces behavioural quiescence On the basis of the observation that nlp-22 mRNA expression cycles during larval development in phase with the cycling of sleep-like behaviour, we hypothesized that it regulates lethargus quiescence. To test this hypothesis, we genetically manipulated nlp-22 expression and observed the effects on quiescence and active behaviour. We first studied the effect of temporal and spatial mis-expression of nlp-22 during the adult stage, when the animals are typically feeding and moving. C. elegans moves by making dorsal and ventral body bends initiated at the anterior end of the animal [23] and feeds by rhythmic pharyngeal contractions called pumps [24] . When we overexpressed nlp-22 using an inducible heat-shock promoter ( Fig. 2a ) during the normally active adult period, we observed quiescence of feeding and locomotion ( Fig. 2b,c , Supplementary Movie 1 , Supplementary Table S1 ). Two hours after heat shock, control animals made 15.9±7.3 (all values presented as mean±s.d.) ( N =15) anterior body bends per min, whereas animals overexpressing nlp-22 made 0.55±1.1 ( N =25) body bends per min ( Fig. 2b ). Wild-type animals and transgenic control animals expressing GFP under the control of a heat-shock promoter pumped 2 h after heat shock at rates of 264.9±17.4 ( N =20) and 273.6±17.5 ( N =20) pumps per min, respectively ( Fig. 2c , Supplementary Table S1 ). Animals carrying the integrated or extrachromosomal Phsp16.2 : nlp- 22 arrays, qnIs142 or qnEx95 , pumped at rates of 18.6±31.1 ( N =37) and 25.2±32.3 ( N =40) per min, respectively, 2 h after heat shock ( Fig. 2c , Supplementary Table S1 ). In the absence of either the signal sequence or the dibasic residues predicted to be necessary for preproprotein cleavage [25] , nlp-22 overexpression no longer promoted behavioural quiescence ( Fig. 2c ), indicating that these features of the protein are important for its biological activity. When we mutated any of the four C-terminal amino acids of the predicted peptide, overexpression of the gene no longer caused quiescence ( Fig. 2c ), indicating that these four amino acids are important for the peptide’s biological function. Nine hours after nlp-22 overexpression, all the animals resumed feeding, indicating that the reduction in behaviour was not due to an injurious effect ( Fig. 2d ). 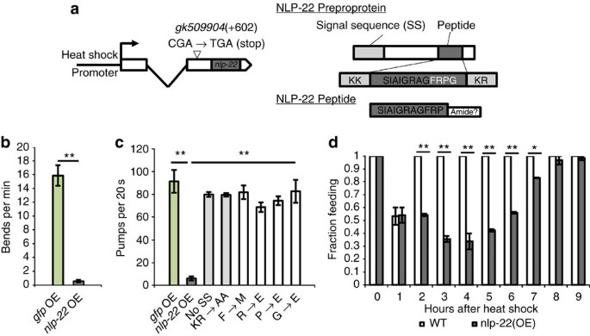Figure 2: NLP-22 induces behavioural quiescence. (a) Gene and protein structure ofnlp-22including overexpression construct. Animals show reduced movement (b) and feeding (c) relative to control animals overexpressing GFP (strain: TJ375), 2.5 h afternlp-22induction. (c) Removing the signal sequence or mutating the KR or FRPG eliminates the ability of NLP-22 to reduce pumping rate (**P<0.0001, Student’s two-tailedt-test,N≥20). (d) Animals overexpressingnlp-22cease pumping, but recover 9 h after heat shock (*P<0.001, **P<0.0001, Fisher’s exact test,N≥20 animals, two trials; Error bars represent s.e.m.). Figure 2: NLP-22 induces behavioural quiescence. ( a ) Gene and protein structure of nlp-22 including overexpression construct. Animals show reduced movement ( b ) and feeding ( c ) relative to control animals overexpressing GFP (strain: TJ375), 2.5 h after nlp-22 induction. ( c ) Removing the signal sequence or mutating the KR or FRPG eliminates the ability of NLP-22 to reduce pumping rate (** P <0.0001, Student’s two-tailed t -test, N ≥20). ( d ) Animals overexpressing nlp-22 cease pumping, but recover 9 h after heat shock (* P <0.001, ** P <0.0001, Fisher’s exact test, N ≥20 animals, two trials; Error bars represent s.e.m.). Full size image NLP-22-induced quiescence resembles lethargus quiescence During lethargus, animals are less responsive to stimuli, a property shared with sleeping vertebrates [12] . In addition, worms in lethargus move backwards more often than non-lethargus worms [26] . Similar to wild-type worms in lethargus, adult worms overexpressing nlp- 22 showed reduced responsiveness to optic or chemical stimulation compared with transgenic control animals that overexpressed GFP ( Fig. 3a ). Under mild heat-shock conditions, in which nlp-22 -overexpressing adult animals were not completely quiescent, they moved backwards more often than control animals ( Fig. 3b ). Thus, overexpression of NLP-22 induces feeding and movement quiescence that is reminiscent of lethargus quiescence. 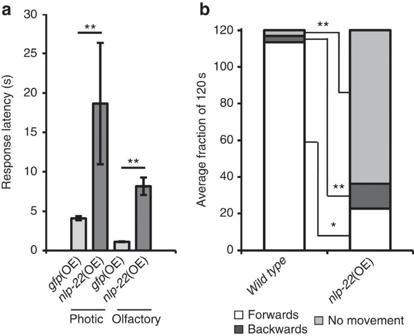Figure 3: Quiescence induced bynlp-22OE resembles lethargus quiescence. (a) Animals that overexpressnlp-22(strain: NQ251) are less responsive to chemical (1-octanol) and optical (blue light) stimulation than control animals that overexpress GFP (strain: TJ375) (**P<0.0001, Student’s two-tailedt-test,N≥20; Error bars represent s.e.m.). (b) Overexpressingnlp-22via a mild heat shock, such that full quiescence is not induced, results in increased backwards movement. White, dark grey and light grey denote forwards, backwards and no movement, respectively. The average fraction of time spent moving forwards or moving backwards in a 120s window fornlp-22overexpressing animals is significantly different from WT worms (*P<0.001. **P<0.0001, Student’s two-tailedt-test,N=20). In addition to the bias for backwards motion,nlp-22overexpressing animals also moved significantly less than WT animals (**P<0.0001, Student’s two-tailedt-test,N=20). Figure 3: Quiescence induced by nlp-22 OE resembles lethargus quiescence. ( a ) Animals that overexpress nlp-22 (strain: NQ251) are less responsive to chemical (1-octanol) and optical (blue light) stimulation than control animals that overexpress GFP (strain: TJ375) (** P <0.0001, Student’s two-tailed t -test, N ≥20; Error bars represent s.e.m.). ( b ) Overexpressing nlp-22 via a mild heat shock, such that full quiescence is not induced, results in increased backwards movement. White, dark grey and light grey denote forwards, backwards and no movement, respectively. The average fraction of time spent moving forwards or moving backwards in a 120s window for nlp-22 overexpressing animals is significantly different from WT worms (* P <0.001. ** P <0.0001, Student’s two-tailed t -test, N =20). In addition to the bias for backwards motion, nlp-22 overexpressing animals also moved significantly less than WT animals (** P <0.0001, Student’s two-tailed t -test, N =20). Full size image NLP-22 is required for proper quiescence during lethargus Our overexpression studies demonstrate sufficiency of nlp-22 for the induction of behavioural quiescence. However, overexpression experiments are likely to result in supra-physiological concentrations of the peptide as well as spatially ectopic expression. Therefore, we proceeded to study a loss of function nlp-22 mutation to ask the question: Is nlp-22 necessary for quiescence? The nlp-22 allele gk509904 has a point mutation that introduces a stop codon before the NLP-22 peptide ( Fig. 2a ); thus, it is likely to fully eliminate nlp-22 function. We measured quiescence in wild-type and nlp-22(gk509904) animals from the active L3 stage through development into adulthood. Total quiescence during L4 lethargus of gk509904 mutants was reduced in comparison with total quiescence of wild-type animals ( Fig. 4a,c and Supplementary Table S2 ). The quiescence defect of gk509904 mutants was rescued by expression of a genomic fragment spanning the nlp-22 locus ( Fig. 4a,c and Supplementary Table S2 ). To test for the functional relevance of the observed RIA gene reporter expression, we expressed nlp-22 double-stranded RNA (dsRNA) to knockdown nlp-22 mRNA specifically in RIA, and, as a control, in the hypodermis. Expression in the RIA neurons but not in the hypodermis reduced lethargus quiescence ( Fig. 4b,c and Supplementary Table S2 ). In addition to reduced quiescence, nlp-22(gk509904) mutants showed enhanced responsiveness to optic sensory stimulation during L4 lethargus quiescence bouts ( Fig. 4d ), demonstrating reduced sleep-like behaviour. Thus, nlp-22 is required for appropriate C. elegans sleep-like quiescence during lethargus. 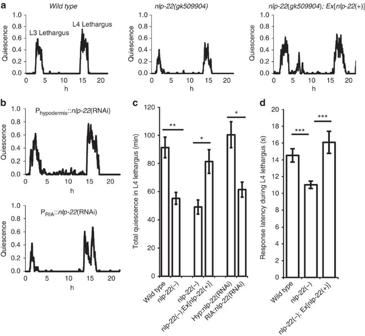Figure 4:nlp-22is required for normal quiescence during lethargus. (a) Fraction of quiescence in a 10-min moving window in a wild-type animal, annlp-22(gk509904)mutant and annlp-22(gk509904) mutant carrying annlp-22genomic rescuing transgene. Thex-axis is hours from the start of recording in the late third larval stage. (b) Quiescence in animals expressing double-strandednlp-22RNA in the hypodermis and in the RIA neurons. Average quiescence (*P<0.05, **P<0.01, ***P<0.001, Student’s two-tailedt-test;N≥10, error bars represent s.e.m.), (c) and response latencies to blue light (d) during fourth larval stage lethargus (***P<0.001, Student’s two-tailedt-test;N≥28 animals, error bars represent s.e.m.). Figure 4: nlp-22 is required for normal quiescence during lethargus. ( a ) Fraction of quiescence in a 10-min moving window in a wild-type animal, an nlp-22(gk509904) mutant and an nlp-22 ( gk509904 ) mutant carrying an nlp-22 genomic rescuing transgene. The x -axis is hours from the start of recording in the late third larval stage. ( b ) Quiescence in animals expressing double-stranded nlp-22 RNA in the hypodermis and in the RIA neurons. Average quiescence (* P <0.05, ** P <0.01, *** P <0.001, Student’s two-tailed t -test; N ≥10, error bars represent s.e.m. ), ( c ) and response latencies to blue light ( d ) during fourth larval stage lethargus (*** P <0.001, Student’s two-tailed t -test; N ≥28 animals, error bars represent s.e.m.). Full size image NLP-22 signals through a PKA-dependent mechanism To determine mechanisms by which nlp-22 induces sleep-like behaviour, we crossed animals carrying nlp-22 overexpression arrays into a subset of the genetic backgrounds that have been previously shown to affect C. elegans quiescence ( kin-2 (ref. 27 ), egl-4 (ref. 12 ) and ceh-17 (ref. 14 )) and into genetic backgrounds known to affect neuropeptide processing or release ( egl-3 (ref. 28 ), egl-21 (ref. 29 ) and unc-31 (ref. 30 )) ( Supplementary Table S1 ). In all cases, but one, the quiescence-inducing effects of nlp-22 overexpression were no different in the mutant background from these effects in the wild-type background. The one observed exception was in kin-2(ce179) mutants, in which the normal inhibition of the catalytic subunits of the cAMP-dependent protein kinase PKA by the regulatory subunits is impaired due to a mutation in the regulatory subunit, resulting in excess activity of the catalytic subunit [31] . Excessive PKA activity causes increased wakefulness in C. elegans and other species [32] . kin-2 mutants are hyperactive [33] , are hyper-responsive to stimuli during lethargus, and show reduced lethargus quiescence [27] . In the kin-2 -mutant background, P hsp16.2 : nlp-22 transgenic animals continued to feed and move from 2.5 to 4.0 h after heat shock ( Fig. 5a,b ). Thus, a reduction in PKA activity is required for NLP-22-induced quiescence. Although kin-2 mutants continued to pump upon nlp-22 overexpression, pumping rates were reduced relative to kin-2- mutant controls ( Supplementary Table S1 ), indicating that either residual kin-2 activity in the mutant analysed is sufficient to reduce PKA activity in response to nlp-22 overexpression or that there are also PKA-independent pathways regulating feeding and locomotion quiescence in response to nlp-22 . 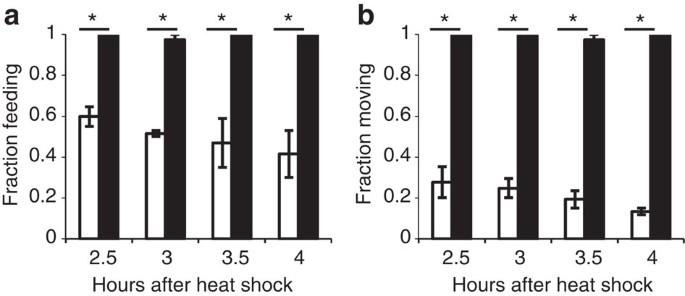Figure 5: NLP-22-induced quiescence requires the protein kinase A subunit KIN-2. Feeding (a) and locomotion (b) quiescence induced bynlp-22overexpression is impaired inkin-2mutants (*P<0.0001, Fisher’s exact test,N>20 animals, 2 trials; error bars represent s.e.m.). Unfilled bars represent animals of genotypeqnIs142(Phsp-16.2:nlp-22;Phsp-16.2:gfp;Pmyo-2:mCherry; unc-119(+)) and filled bars represent animals of genotypeqnIs142; kin-2(ce179)X. Figure 5: NLP-22-induced quiescence requires the protein kinase A subunit KIN-2. Feeding ( a ) and locomotion ( b ) quiescence induced by nlp-22 overexpression is impaired in kin-2 mutants (* P <0.0001, Fisher’s exact test, N >20 animals, 2 trials; error bars represent s.e.m.). Unfilled bars represent animals of genotype qnIs142 (P hsp-16.2:nlp-22; P hsp-16.2:gfp; P myo-2:mCherry; unc-119 (+)) and filled bars represent animals of genotype qnIs142; kin-2 ( ce179 )X. Full size image The RIAs have quiescence- and movement-promoting properties Because the RIA neurons express the somnogenic peptide NLP-22, we hypothesized that they are quiescence-promoting neurons. To test this hypothesis, we used the strain VM1345, which expresses the cell death gene interleukin-lβ-converting Enzyme ( ICE ) [34] , [35] , [36] in the RIA neurons. Because of the incomplete penetrance of the RIA ablation phenotype in VM1345, in a subset of the animals only one of the two RIAs died. We compared L4 lethargus quiescence in animals lacking one or two RIAs to a control transgenic strain with both RIA neurons intact. There was a significant reduction in lethargus quiescence in animals lacking both RIA neurons ( Fig. 6a ), consistent with the hypothesis that RIA neurons promote quiescence. Animals lacking only one of the RIA neurons also showed a small but significant reduction in L4 lethargus quiescence compared with control transgenic animals ( Fig. 6a ). 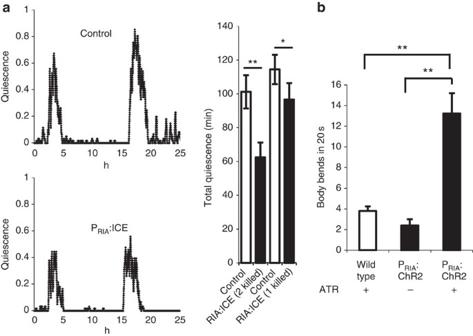Figure 6: The RIA neurons have both quiescence- and movement-promoting functions. (a) Genetic ablation of the RIA interneurons using the cell death protein ICE (strain:VM1345) decreases quiescence during lethargus compared with control transgenic animals (strain: NQ156). The traces depict the fraction of quiescence in a 10-min time interval. The top trace is of a control animal of genotypelin-15(n765ts)X;qnEx48(Pins-4:gfp:PEST;lin-15(+)), and the bottom trace is of an experimental animal of genotypelin-15(n765ts)X;akEx211(Pglr-3:gfp; Pglr-3:ICE;lin-15(+)). Total quiescence during L4 lethargus is lower in experimental animals lacking either one or both RIA neurons than in control animals to which they were paired (*P<0.05, **P<0.001, Student’s two-tailedt-test,N≥9; error bars represent s.e.m.). (b) Optogenetic stimulation of the RIA neurons promotes movement during lethargus. WT animals grown on all-transretinal (ATR) and PRIA:ChR2 worms grown either in the absence or presence of ATR, were identified as they entered L4 lethargus, transferred to a new plate and were unperturbed for 15 min until they became quiescent. Body bends were counted for 1 min after a 15-s exposure of quiescent animals to blue light. PRIA:ChR2 animals on ATR moved significantly more than control animals (*P<0.05, **P<0.001, Student’s two-tailedt-test, WT (N=15), No ATR vs ATR (N≥20); error bars represent s.e.m.). Figure 6: The RIA neurons have both quiescence- and movement-promoting functions. ( a ) Genetic ablation of the RIA interneurons using the cell death protein ICE (strain:VM1345) decreases quiescence during lethargus compared with control transgenic animals (strain: NQ156). The traces depict the fraction of quiescence in a 10-min time interval. The top trace is of a control animal of genotype lin-15 ( n765ts )X; qnEx48 (P ins-4 : gfp : PEST ; lin-15 (+)), and the bottom trace is of an experimental animal of genotype lin-15 ( n765ts )X; akEx211 (P glr-3 : gfp ; P glr-3 :ICE; lin-15 (+)). Total quiescence during L4 lethargus is lower in experimental animals lacking either one or both RIA neurons than in control animals to which they were paired (* P <0.05, ** P <0.001, Student’s two-tailed t -test, N ≥9; error bars represent s.e.m.). ( b ) Optogenetic stimulation of the RIA neurons promotes movement during lethargus. WT animals grown on all- trans retinal (ATR) and P RIA :ChR2 worms grown either in the absence or presence of ATR, were identified as they entered L4 lethargus, transferred to a new plate and were unperturbed for 15 min until they became quiescent. Body bends were counted for 1 min after a 15-s exposure of quiescent animals to blue light. P RIA :ChR2 animals on ATR moved significantly more than control animals (* P <0.05, ** P <0.001, Student’s two-tailed t -test, WT ( N =15), No ATR vs ATR ( N ≥20); error bars represent s.e.m.). Full size image This neuron ablation experiment supports the notion that the RIA neurons promote sleep-like behaviour. However, removing the neuron by genetic ablation is a chronic manipulation that removes all functions of the neurons, including both those related to rapid signalling via membrane voltage changes as well as chronic signalling via mechanisms independent of membrane voltage. To test whether acute depolarization of the RIA neurons also induces quiescence, we made transgenic animals expressing the blue light-activated cation channel channelrhosopsin-2 (ChR2) [37] in the RIA neurons. We optogenetically depolarized the RIA neurons during the active L4 stage as well as during L4 lethargus. Animals carrying the ChR2 transgene in the RIA neurons were cultivated in the absence ( N =4) or presence ( N =7) of the ChR2 co-factor all- trans retinal (ATR) and followed for 8 h during the active L4 stage. The animals were exposed to blue light for 15 s every 30 min and monitored for locomotion and feeding quiescence. Stimulating the RIA neurons during the active L4 stage caused no induction in behavioural quiescence. In contrast, optogenetic depolarization of the RIA neurons during L4 lethargus had a locomotion-stimulating effect. Compared with control animals lacking the ChR2 transgene and with control animals carrying the transgene, but lacking ATR, stimulation of the RIA neurons increased movement during lethargus ( Fig. 6b ). Thus, acute depolarization of the RIA neurons during lethargus promotes wake-like behaviour. We conclude that the RIA neurons have both quiescence-promoting effects, revealed by chronic ablation, and wake-promoting effects, revealed by acute depolarization. Thus, the RIA neurons are complex regulators of lethargus quiescence with both movement- and quiescence-promoting roles. NLP-22 is structurally similar to mammalian Neuromedin S The NLP-22 predicted peptide has a glycine at its C-terminus. In previous analyses, C. elegans neuropeptides with a C-terminal glycine have been shown to be deglycinated and then amidated during peptide maturation [38] . Hence, NLP-22 has been termed an FRPamide peptide, corresponding to a Phenylalanine(F)-Arginine(R)-Proline(P) motif [19] ( Fig. 2a ). Using the alignment program Muscle (version 3.7) [39] on the Phylemon 2.0 platform [40] , we found that the predicted NLP-22 neuropeptide in C. elegans is nearly identical to orthologous proteins of four other nematodes (Fig. 8a), indicating strong functional selection on the neuropeptide sequence. Comparing the NLP-22 neuropeptide with human neuropeptides, we noted similarities with neuromedin S (NMS). Both the NLP-22 and NMS peptides are located near the C-terminus of the preproprotein (Fig. 8b) and are composed of the dipeptide Glycine(G)-Arginine(R) located in the middle of the peptide and the tripeptide FRP located at or close to the C-terminus (Fig. 8b). To further compare NLP-22 to NMS, we used the peptide structure algorithm Pep-Fold [41] , which predicts the three-dimensional structures of small peptides. Pep-Fold predicts that NLP-22 forms an anti-parallel beta-sheet where the conserved GR dipeptide is within the loop, and the C-terminal FRP is near the end of the second sheet (Fig. 8c). Interestingly, human NMS is predicted to form the same general structure (Fig. 8c). These structural similarities suggest that NLP-22 and NMS may be orthologous peptides. Wake-promoting neuropeptides such as hypocretin/orexin in vertebrates and PDF in Drosophila have well-defined roles as modulators of sleep/wake as an output of the circadian clock [9] . However, few physiologically relevant sleep-promoting peptides have been identified [3] , [5] , [42] , and their relationship to the circadian clock is poorly understood. We have identified NLP-22 as a C. elegans somnogenic peptide. NLP-22 activity is partially regulated at the level of mRNA abundance in response to a LIN-42/PER-based larval clock, suggesting that similar somnogens may function as the output to the PER-based circadian clock in other species. How might LIN-42 be regulating nlp-22 expression? Drosophila PER acts as a cell autonomous negative regulator of transcription of genes that are positively regulated by the transcription factors CLK and CYC [20] . In response to ectopic expression of LIN-42, we observed nlp-22 mRNA induction only after 6–8 h, which is delayed relative to a typical heat-shock response [43] . If LIN-42 were functioning in C. elegans similarly to PER function in Drosophila , then LIN-42 could repress transcription of a gene that negatively regulates nlp-22 expression in the same cell. Alternatively, the interaction could be non-cell autonomous. In support of a possible non-cell autonomous interaction, restoration of LIN-42 in the hypodermis of lin-42 mutants partially rescues the asynchronous nature of lethargus quiescence [17] yet nlp-22 is expressed outside the hypodermis, in the RIA interneurons. Even if LIN-42 were regulating nlp-22 expression directly, then it must also regulate other genes, as nlp-22 mutants do not show other phenotypes observed for lin-42 mutants such as heterochronic defects, slow growth and moulting defects [17] , [44] . What is the role of the RIA interneurons during lethargus quiescence? The RIAs are a highly connected pair of interneurons that are required for thermotaxis [45] and aversive/associative learning [35] , [46] , [47] , [48] . Our data suggest that the RIAs also control sleep-like behaviour. Surprisingly, our experiments revealed both quiescence- and movement-promoting functions for the RIA neurons. Our results suggest that the RIAs release two factors with different behavioural effects: the neuropeptide NLP-22, which decreases PKA activity in an unidentified cell type ( Fig. 7 ) to promote quiescent behaviour and an unknown transmitter, which promotes movement. As acute depolarization of RIA promotes movement and not quiescence, the mechanism of NLP-22 release may be different from that of the movement-promoting transmitter. NLP-22 release may be regulated by secondary messengers independently from the membrane voltage. For example, a local calcium increase without membrane potential change could promote NLP-22 secretion without affecting the release of wake-promoting factor. Consistent with this possibility, the RIA neurons show subcellular compartmentalization of intracellular calcium levels [49] . In addition, NLP-22 availability is regulated at least partially at the level of mRNA abundance. Regardless of the explanation for these results, they highlight both the limitation of relying on ablation alone to infer neuron function and the benefit of using acute optogenetic activation to understand neuronal function. 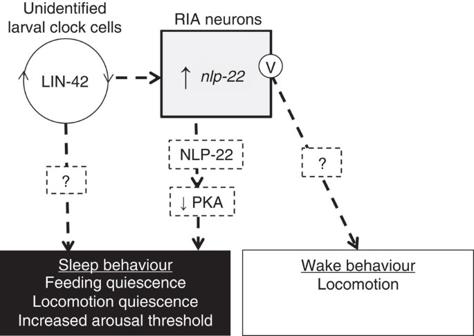Figure 7: Model for role ofnlp-22and RIA in sleep-like quiescence regulation. LIN-42 functions in as yet unidentified larval clock cells to regulate nlp-22 expression as well as other quiescence-regulatory factors. Release of NLP-22 neuropeptide promotes sleep-like behaviour via a reduction in protein kinase A (PKA) activity. RIA membrane depolarization (marked with the letter V) results in the release of an unidentified wake-promoting neurotransmitter. Figure 7: Model for role of nlp-22 and RIA in sleep-like quiescence regulation. LIN-42 functions in as yet unidentified larval clock cells to regulate nlp-22 expression as well as other quiescence-regulatory factors. Release of NLP-22 neuropeptide promotes sleep-like behaviour via a reduction in protein kinase A (PKA) activity. RIA membrane depolarization (marked with the letter V) results in the release of an unidentified wake-promoting neurotransmitter. Full size image We have shown that NLP-22 and mammalian NMS are structurally similar ( Fig. 8 ). In addition, NLP-22 and NMS show intriguing functional similarities. NMS shows a diurnal pattern of mRNA expression and is predominately expressed in a small set of central nervous system neurons in the suprachiasmatic nucleus [7] . Like NMS, NLP-22 cycles its expression, only as the output of a larval-based clock, and like NMS, NLP-22 is selectively expressed, in a single-neuron pair, the RIAs ( Fig. 1c ). Although the suprachiasmatic nucleus is well known as the master circadian clock pacemaker [50] , a role for the RIAs in regulating the analogous larval clock in C. elegans has not been reported. The RIAs are required for C. elegans memory behaviours [35] , [48] , behaviours that in mammals are sensitive to the sleep-wake history of the animal [51] . 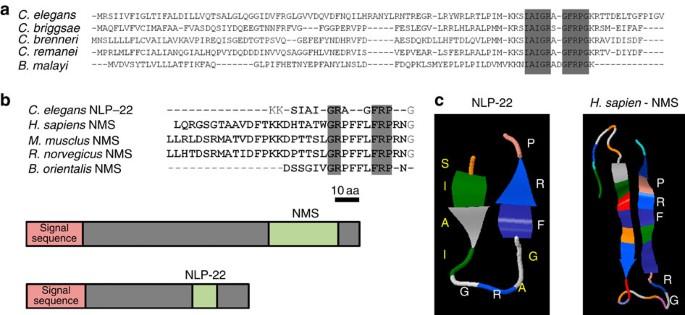Figure 8: NLP-22 is similar to Neuromedin S. (a) Alignment of NLP-22 preproprotein with orthologs from four nematode species. High conservation (grey box) is observed in the predicted neuropeptide sequence. (b) Amino-acid sequence similarities (grey boxes) between NLP-22 and vertebrate Neuromedin S peptides. The preproprotein structure of human Neuromedin S and NLP-22 is also shown. Each has an N-terminal signal sequence and a single, C-terminal peptide. The preproprotein is drawn to scale (Bar=10 amino acids). (c) Predicted structures of NLP-22 and of NMS. The conserved GR dipeptide and FRP tripeptide motifs are shown in white. Figure 8: NLP-22 is similar to Neuromedin S. ( a ) Alignment of NLP-22 preproprotein with orthologs from four nematode species. High conservation (grey box) is observed in the predicted neuropeptide sequence. ( b ) Amino-acid sequence similarities (grey boxes) between NLP-22 and vertebrate Neuromedin S peptides. The preproprotein structure of human Neuromedin S and NLP-22 is also shown. Each has an N-terminal signal sequence and a single, C-terminal peptide. The preproprotein is drawn to scale (Bar=10 amino acids). ( c ) Predicted structures of NLP-22 and of NMS. The conserved GR dipeptide and FRP tripeptide motifs are shown in white. Full size image The central nervous system administration of NMS into mammals and birds inhibits feeding behaviour [52] , [53] , [54] , [55] . NLP-22 overexpression causes an almost complete block of feeding in C. elegans ( Fig. 2 ). The central nervous system administration of NMS in rats causes an inhibition of locomotion and a phase shift of the circadian behavioural rhythm [7] . NLP-22 overexpression causes behavioural quiescence during the normally active adult stage ( Fig. 2 ). Our work predicts effects of NMS on sleep behaviour, but to our knowledge this has not yet been tested. Although there are functional and structural similarities between NLP-22 and NMS, there are also clear differences. Mammalian NMS has a highly conserved C-terminal RN motif that is not present in C. elegans NLP-22. When we overexpressed human NMS(17–33), which contains the 17 C-terminal amino acids of NMS including the amino acids conserved with NLP-22 and which is predicted to form a similar three-dimensional structure as NLP-22 and full-length NMS ( Supplementary Fig. S2a ), we did not observe behavioural quiescence in C. elegans ( Supplementary Fig. S2b ). Furthermore, we could not identify genes coding for proteins predicted to be processed into NLP-22 or NMS-like peptides in the genomes of insects or fish. Finally, loss of function of each of four G-protein-coupled receptors that are weakly similar to a mammalian NMS receptor [56] did not suppress the NLP-22-induced quiescence ( Supplementary Table S1 ). Neuropeptides and neuropeptide receptors often show co-evolution, leading to difficulty in identifying homologues across phyla [57] . Thus, future additional data, including the identification of the NLP-22 post-synaptic signalling pathway, will be required to determine whether NLP-22 and NMS are true homologues. In summary, our work defines the first role for a somnogenic neuropeptide in C. elegans and identifies a pair of neurons, the RIAs, in the regulation of C. elegans sleep-like behaviour. Although C. elegans sleep-like behavioural research is still in its nascent stage, the simplicity of this model animal’s nervous system combined with recent progress in the identification of cells involved in sleep-like behavioural regulation [13] , [14] , [15] , [58] , [59] holds promise for rapid future progress in delineating the genes and circuits regulating sleep and wake. Cultivation methods and strains Animals were cultivated on NGM agar and, unless noted otherwise, were fed the OP50 E. coli derivative strain DA837 (ref. 60 ). All experiments were performed on hermaphrodites. The following strains were used in this study: N2 (Bristol), EG4322 ttTi5605 II; unc-119(ed3)III , TJ375 gpIs1(Phsp-16.2::gfp) , NQ156 lin-15 ( n765ts )X; qnEx48 (P ins-4 : gfp : PEST ; lin-15 (+)), NQ216 unc-119(ed3)III;qnEx95 (P hsp-16.2 :: nlp-22; Pmyo-2:mCherry; unc-119(+) ), IB16 ceh-17 ( np1 )I, NQ230 ceh-17 ( np1 )I; qnEx95 , NQ235 nmur- 4( ok1381 )I; qnEx95 , NQ250 qnIs101(Pnlp-22 : nlp-22 : gfp ; Pmyo-2:mCherry ; unc-119 (+)), NQ251 qnIs142(Phsp-16.2:nlp-22 ; Phsp-16.2 : gfp ; Pmyo-2 :mCherry, unc-119 (+)), DA509 unc-31(e928)IV , NQ256 unc-31 ( e928)IV;qnEx95 , NQ266 unc-119 ( ed3 )III; qnEx128 (P nlp-22 :gfp: nlp-22 ; Pmyo-2 : mCherry ; unc-119 (+)), NQ269 unc-119 ( ed3 )III; qnEx131 (P hsp-16.2 : nlp-22 (No Signal Sequence); P myo-2 :mCherry; unc-119(+) ), NQ270 unc-119 ( ed3 ) III;qnEx132(Phsp-16.2 : nlp-22 (No Signal Sequence); P myo-2 :mCherry; unc-119 (+)), NQ274 nmur- 1( ok1387 )X; qnEx95 , NQ275 nmur-3 ( ok2295 )X; qnEx95 , NQ282 unc-119 ( ed3 )III; qnEx139(Phsp-16.2 : nlp-22 (No Signal Sequence); Pmyo-2 : mCherry ; unc-119 (+)), NQ285 nmur-2 ( ok3502 )II; qnEx95 , NQ305 sid-1 ( pk3321 )V; qnIs137 (P dpy-7:nlp-22(RNAi); Pmyo-2:mCherry; unc-119(+) ), NQ314 unc-119 ( ed3 )III; qnEx160(Phsp-16.2 : nlp-22 (KR → AA); Pmyo-2 : mCherry ; unc-119 (+)), KP1873 egl-3(nu349)V , NQ319 egl-3 ( nu349 )V; qnEx95 , KP2018 egl-21(n476)IV , NQ320 egl-21 ( n476 )IV; qnEx95 , MT1074 egl-4 ( n479 )IV , NQ321 egl-4 ( n479 )V; qnEx95 , NQ333 unc-119 ( ed3 )III; qnEx162 (P nlp-22 :Intron: gfp ; P myo-2 :mCherry; unc-119 (+)), NQ367 unc-119 ( ed3 )III; qnEx178 (P hsp-16.2 : nlp-22 (KR → AA); Pmyo-2:mCherry ; unc-119 (+)), NQ374 unc-119 ( ed3 )III; qnEx185 (P hsp-16.2 : nlp-22 (FRPG → MRPG); P myo-2 :mCherry; unc-119 (+)), NQ375 unc-119 ( ed3 )III; qnEx186 (P hsp-16.2 : nlp-22 (FRPG → MRPG); P myo-2 :mCherry; unc-119 (+)), NQ376 sid-1 ( pk3321 )V; qnIs157 ( glr-3:nlp-22(RNAi); myo-2:mCherry; unc-119(+) ), NQ378 unc-119 ( ed3 )III; qnEx187 (P hsp-16.2 : nlp-22 (FRPG → FEPG); P myo-2 :mCherry; unc-119 (+)), NQ379 unc-119 ( ed3 )III; qnEx187 (P hsp-16.2 : nlp-22 (FRPG → FEPG); P myo-2 :mCherry; unc-119 (+)), NQ383 unc-119 ( ed3 )III; qnEx192 (P hsp-16.2 : nlp-22 (FRPG → FRPE); P myo-2 :mCherry; unc-119 (+)), NQ392 unc-119 ( ed3 )III; qnEx188 (P hsp-16.2 : nlp-22 (FRPG → FREG); P myo-2 :mCherry; unc-119 (+)), NQ393 unc-119 ( ed3 )III; qnEx189 (P hsp-16.2 : nlp-22 (FRPG → FREG); P myo-2 :mCherry; unc-119 (+)), NQ448 unc-119 ( ed3 )III; qnEx224 (P glr-3 :ChR2::YFP (Regular)+ unc-122 :gfp+ unc-119 (+)) ARF240 aaaIs1 ( Phsp-16::lin-42a::unc-54utr; P myo-2:dsRed ), NQ596 nlp-22 ( gk509904 )X, NQ603 nlp-22 ( gk509904 )X; qnEx311 ( nlp-22 (+); Pmyo-2:Cherry ), KG532 kin-2(cd179 )X, NQ606 kin-2 ( cd179 )X; qnIs142 ; VC40199 nlp-22 ( gk509904 )X; NQ667 kin-2 ( ce179 )X; qnEx95 , NQ668 egl-4 ( n479 )IV; qnIs142 , NQ670 qnEx95 , VM1345 lin-15 ( n765ts )X; akEx211 (P glr-3 : gfp ; P glr-3 :ICE; lin-15 (+)), RB1288 nmur-1 ( ok1387 )X, RB2526 nmur-2 ( ok3502 )II, VC1974 nmur-3 ( ok2295 )X, RB1284 nmur-4 ( ok1381 )I. Molecular biology and transgenesis All DNA constructs were made using overlap-extension PCR [61] . In brief, to fuse two or more DNA fragments, we amplified (Herculase Enhanced DNA Polymerase, Agilent Technologies) the individual DNA fragments with oligonucleotides that included 5′-extensions complementary to the fusion target. Individually amplified DNA fragments were then mixed without primers in the presence of DNA polymerase in order to anneal and extend the fused product. The fused product was purified (QIAquick PCR Purification Kit, Qiagen) and amplified using nested primers. The size of the final PCR product was verified by performing gel electrophoresis [61] . Oligonucleotides used for making these constructs are listed in Supplementary Table S3 . For nlp - 22 overexpression, the promoter of hsp-16.2 was amplified from the vector pPD49.83 (obtained from Addgene) and fused to the genomic sequence of nlp-22 (+1 to +1,451) (where nucleotide number refers to the nucleotide position relative to the start site of translation). Both the extrachromosomal array, qnEx95 , and the integrated array, qnIs142 , were analysed in each behavioural assay. The mutated nlp-22 overexpression constructs (No signal sequence (SS), KR → AA, FRPG → MRPG, FRPG → FEPG, FRPG → FREG, FRPG → FRPE) were created by introducing the desired mutations by overlap-extension PCR using oligonucleotide 5′-extensions that encoded the amino-acid changes [61] . Each mutated fused PCR product was cloned into a pCR2.1-TOPO TA Vector (Invitrogen) and then sequenced to verify that the intended mutation but no other mutation was introduced. At least two and often three independent lines were analysed for each behavioural analysis. To make a fusion protein in which GFP is at the C-terminus of the NLP-22 protein, the genomic sequence of nlp-22 (−450 to +701) was fused in frame to gfp followed by the unc-54 3′UTR, which was amplified from the vector pPD95.75 (Addgene). To make a fusion in which GFP is at the N-terminus of the NLP-22 protein, the promoter (−450 to +3) of nlp-22 was fused to the coding sequence of GFP amplified from pPD95.75 only excluding the stop codon and fused in frame to the genomic sequence of nlp-22 (+1 to +701), which included the nlp-22 3′UTR. The transcriptional reporter for nlp-22 ( Pnlp-22:Intron:gfp ) was made by fusing the promoter of nlp-22 (−450 to +3) to the coding sequence of GFP, amplified from pPD95.75 and replacing one of the synthetic introns of gfp with the intron of nlp-22 (+85 to +481). To drive expression of nlp-22 dsRNA in the RIA neurons, the promoter of glr-3 (−5,500 to −1) was fused to the genomic sequence of nlp-22 spanning the region +13 to +653 in the sense orientation, and, in a separate reaction, to the nlp-22 genomic sequences spanning the same nucleotides in the anti-sense orientation. These constructs lack a start codon and 3′UTR of nlp-22 . To drive expression of nlp-22 dsRNA in the hypodermis, the promoter of dpy-7 (−417 to −1) amplified from N2 genomic DNA was fused to nlp-22 sense and anti-sense DNA. The genomic rescuing fragment of nlp-22 spanned from −450 to +1,451 relative to the nlp-22 start codon. To overexpress Neuromedin S (17–33) (Phoenix Pharmaceuticals), we replaced the coding sequence for the nlp-22 peptide with the coding sequence for Neuromedin S (17–33) and fused the nlp- 22-NMS(17–33) chimeric sequence to the heat-shock promoter. Transgenic animals were created by microinjection [62] using a Leica DMIRB inverted DIC microscope equipped with an Eppendorf Femtojet microinjection system. EG4322 animals were injected with 25–50 ng μl −1 of each construct in combination with 5 ng μl −1 pCFJ90 (P myo-2:mCherry ), with 50–100 ng μl −1 of P unc-122 :gfp or pCFJ104 (P rab-3: : mCherry ) and pCFJ151 ( unc-119 (+)) up to a total concentration of 150 ng μl −1 . To make the nlp-22 RNAi strains, 25 ng μl −1 of nlp-22 (sense) and nlp-22 (anti-sense) were injected together with the transgenesis markers pCFJ90 and pCFJ151. For behavioural experiments using transgenic animals carrying extrachromosomal arrays, at least two distinct lines were analysed. In most cases, quantitative behavioural analysis was performed only on one of these transgenic lines, but in all cases the other line(s) gave the same qualitative result. The integrated transgenes qnIs101 , 137 , 142 and 157 were constructed by UV irradiation of the extrachromosomal transgenes qnEx101 , 137 , 142 and 157 (ref. 63 ). A mix of ~100 L4 and adult transgenic animals were placed in a Spectrolinker XL-1500 UV Crosslinker (Spectronics Corporation) and exposed to 30,000 μJ cm −2 of ultraviolet light. Irradiated animals were plated at a density of five animals per plate and grown for multiple generations. Integrants were identified as those that produced 100% transgenic progeny. Each integrated strain was out-crossed to the wild-type strain a minimum of three times before analysis. The strain VC40199 containing the nlp-22 ( gk509904 ) X allele was produced by the million mutation project [64] and obtained from the Caenorhabditis Genetics Consortium. The CGA to TGA mutation in nlp-22 reported for this strain was verified by sequencing a genomic PCR fragment, which was PCR-amplified using the primers oNQ552 and oNQ534 ( Supplementary Table S3 ). The strain NQ596 nlp-22 ( gk509904 ) X was generated by crossing the strain VC40199 to N2 males and then crossing resultant males back to VC40199. This procedure was repeated four times. A twitcher phenotype, which was present in VC40199 animals, was not present in the out-crossed NQ596 animals. Overexpression analysis For all overexpression experiments, animals carrying arrays with inducible heat-shock promoters were grown to young adulthood at 20 °C, transferred to the surface of NGM agar 6-cm diameter plates fully seeded with a lawn of DA837 E. coli bacteria, wrapped in Parafilm and immersed in a 33 °C water bath for 30 min. Heat-shocked animals were placed at 20 °C before analysis. Pharyngeal pumping and body bends were counted during 20 s and 1 min intervals, respectively, two hours after heat-shock. Arousal threshold was determined by measuring the latency to respond to exposure to blue light [65] or exposure to a hair dipped in a freshly prepared mixture of 30% octanol and 70% ethanol [66] . Response to octanol was defined as backwards movement of the magnitude corresponding to one-third of the worm’s length. Response to blue light was defined as movement (either forward or backwards) of magnitude equal to one-half of the animal’s body length. Arousal threshold assays of nlp-22 mutants and nlp-22 mutants carrying a rescuing transgene were performed by an investigator who was blinded to genotype. The blinding was set up by a colleague without the use of a computer randomization program. It was impossible to blind the investigator to the genotype of the nlp-22 (OE) transgenic animals because these animals were extremely quiescent and retained excessive eggs. In experiments designed to assess the effects of mild overexpression of nlp-22 on direction of locomotion, animals were analysed 1 h after a 15 min 33 °C heat exposure. Behaviour was assessed on an agar surface devoid of bacteria. During a 120-s period, we measured with a hand-held timer the total time spent moving forwards as well as the total time spent moving backwards. The average of 20 experimental animals expressing Phsp16.2:nlp-22 ( qnIs142 ) was compared with the average of 20 control N2 animals. Imaging of fluorescence For GFP and differential interference contrast imaging, animals were mounted on 5% agar pads, immobilized with 15 mM levamisole and observed through a × 63 or × 100 objective lens on a Leica DM5500B microscope. Leica LAS software was used to capture images. Quiescence measurements For automated measurements of lethargus quiescence, we placed single larva in moulded, concave polydimethylsiloxane (PDMS) wells of diameter 3 mm and depth 2.5 mm, filled with 15 μl of NGM agar and seeded with DA837 bacteria. In each experiment, we placed one experimental and one control animal into two adjacent wells, and the PDMS was then placed on a Diagnostics Instruments microscope base and illuminated for bright-field microscopy, using white light supplied to the base with a fibre optic cable from a Schott DCR III light source. A camera (659 × 494 pixels, scA640-70fm, Basler Vision Technologies) mounted on a Zeiss Stemi 2000 stereomicroscope captured an image with an 8-bit grayscale of both wells every 10 s. At this magnification and our camera acquisition setting, the spatial resolution was 12.5 micrometers per pixel. To quantify quiescence, we monitored animals for time a period between 12 and 48 h and used a machine vision frame subtraction principle to identify 10-s epochs of behavioural quiescence [12] , [27] , [67] . Recordings were performed in an environmental room at 19±2 °C. In comparison with conditions used in previous quiescence measurements, the room temperature was lower and pixel resolution was reduced, leading to quiescence measurements that were greater than those previously reported [12] . For each experimental condition, quiescence of at least six animals was measured because we previously found this number to be sufficient to detect a difference in quiescence [12] . For most conditions, 9–11 animals were used. Data were discarded if the temperature of the room exceeded 21 °C due to equipment malfunction or if one of the two worms burrowed in the agar. Quiescence data from VM1345 were discarded when, upon inspection with epifluorescence, we determined that neither RIA had died. We censored 12% of the VM1345 data for that reason. qPCR L2 or L3 worms were picked to fresh plates seeded with DA837 bacteria and allowed to enter lethargus. We identified worms in L2 or L3 lethargus, using a Leica MZ16 stereomicroscope, by an absence of locomotion and feeding. A subset of worms was collected for RNA isolation in either L2 or L3 lethargus, whereas the remaining animals were allowed to mature for additional durations before collecting. The experiment was performed at 25 °C to speed development. L4 lethargus animals were similarly identified by first transferring mid L4 animals to a fresh agar dish seeded with DA837 and then collecting animals that had stopped moving and feeding. To test lin-42 -dependent induction of nlp-22 mRNA, ARF240 first day adult animals, which were cultivated at 15 °C, were submersed while housed on an NGM agar surface fully seeded with bacteria in a 33 °C water bath for 30 min and then recovered at 25 °C. Control N2 animals were treated identically. RNA was collected before heat-shock treatment and at 4, 6 and 8 h after the end of the heat treatment. Total RNA was collected from each population using an RNAeasy mini kit (Qiagen), and cDNA was synthesized using the SuperScript one-step RT-PCR system (Invitrogen). We performed three or more biological replicates in each experiment, and for each biological replicate we used the average of two technical real-time PCR replicates. Real-time PCR was performed using Taqman Gene Expression Mastermix on an Applied Biosystems 7500 platform at the core services within the Penn Center for AIDS Research, an NIH-funded program (P30 AI 045008). Oligonucleotides used for the real-time PCR analysis were purchased from IDT, and their sequences are shown in Supplementary Table S3 . Relative mRNA was determined by the delta-delta method [68] by normalization to the expression of the gene pmp-3 (ref. 69 ). How to cite this article: Nelson, M. D. et al. The neuropeptide NLP-22 regulates a sleep-like state in Caenorhabditis elegans . Nat. Commun. 4:2846 doi: 10.1038/ncomms3846 (2013).